Bethe-hole polarization analyser for the magnetic vector of light The nature of light as an electromagnetic wave with transverse components has been confirmed using optical polarizers, which are sensitive to the orientation of the electric field. Recent advances in nanoscale optical technologies demand their magnetic counterpart, which can sense the orientation of the optical magnetic field. Here we report that subwavelength metallic apertures on infinite plane predominantly sense the magnetic field of light, establishing the orientation of the magnetic component of light as a separate entity from its electric counterpart. A subwavelength aperture combined with a tapered optical fibre probe can also serve as a nanoscale polarization analyser for the optical magnetic field, analogous to a nanoparticle sensing the local electric polarization. As proof of its functionality, we demonstrate the measurement of a magnetic field orientation that is parallel to the electric field, as well as a circularly polarized magnetic field in the presence of a linearly polarized electric field. The orientation of the electric field has been considered as the light vector ever since Wiener's classic experiments in 1890 showed that the electric field of light initiates photochemical reactions on a photographic film [1] , [2] . The electric field direction of light can be sensed by existing polarizers and the electric field alone has been sufficient to describe the polarization of optical fields, as electric and magnetic fields are usually perpendicular and equal in strength in free space (Gaussian units). On the other hand, for optical fields close to charges and current sources in the quasistatic limit involving evanescent wavevector components, electric and magnetic fields are neither perpendicular nor equal in strength to each other. In these quasistatic cases, which are characteristic of optical fields on nanometre length scales, a magnetic field orientation as a separate entity from its electric counterpart is required for a complete description of the local optical field. The concept of magnetic field polarization is particularly relevant, as recent advances in optical technologies such as plasmonics [3] , [4] , [5] , [6] , negative index metamaterials [7] , [8] , [9] , [10] , [11] , artificial structures with large magnetic dipole moments [12] , [13] , optical antennas and circuits [14] and subwavelength optics [15] , [16] , [17] , [18] , [19] , [20] , [21] , [22] , [23] , [24] , [25] , [26] , [27] have revived the idea that the magnetic field of light is an equally important component of the light vector. Detection of the optical magnetic field, using a subwavelength aperture [15] , [16] , [17] , [18] , on metallic probes, has been achieved. An alternative method is to perform a curl operation on the measured electric field [20] , [21] , [22] to deduce the magnetic field. It has also been shown that a subwavelength aperture on metallic probe tip can induce the magnetic interaction with photonic crystal nanocavity [28] . However, a direct method for determining the unknown magnetic field orientation is yet to be achieved; we need a magnetic polarizer at the optical frequency. Here we show that a metallic circular nanoscale aperture is a magnetic scatterer in complete agreement with Bethe's theoretical analysis on diffraction by a circular aperture [29] , allowing the magnetic field direction to be determined, independent of the electric field direction. This structure is, therefore, a device that functions as a polarization analyser for the magnetic field component of light. We demonstrate that a circular aperture on a flat-bottomed metallic tip is also a polarization analyser for the optical magnetic field, which we use to identify an unusual polarization configuration at which the local magnetic and electric field components of light are parallel to each other, made possible by the interference of two counter-propagating plane waves with orthogonal polarizations. Bethe's single hole determines magnetic field orientation Time-varying magnetic fields induce Eddy currents in metals, which is the principle behind induction heating and welding, as well as metal detection. When light is incident on a subwavelength aperture in a metallic film with a large dielectric constant, the small size of the aperture and the large dielectric constant of the metal result in strong evanescent fields in this quasistatic regime. The tangential magnetic field enters the subwavelength hole with a certain distortion ( Fig. 1a ), with its amplitude at the centre of the aperture equal to that of the incident field. In contrast, the tangential electric field is primarily reflected, its influence being much weaker on both sides of the plane and inside the hole ( Fig. 1b ). Therefore, the scattering properties of an aperture in a metal film are mainly determined by the incident magnetic field-inducing surface currents, which in turn function as a source for far-field radiation [29] , [30] . It should be noted that the magnetic field-dominated scattering process is generally possible with non-circular apertures, but for the present study, a circular hole has been chosen for clarity [31] . 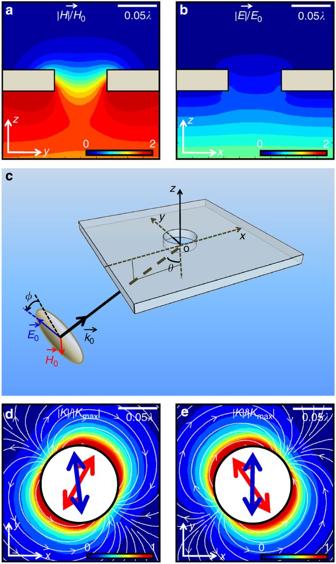Figure 1: Calculated field and current distributions around a subwavelength hole. The metal film has been assumed to be a near-perfect electric conductor with a hole diameter of 0.08λand a thickness of 0.02λ. (a,b) Normalized electric and magnetic field strength distribution with the normal incidence (,), respectively. (c) Schematic of setup with an oblique incidence (θ≠0°)in thexzplane, with the polarization angleφ. (d,e) Surface current distribution on the exit side of the hole forφ=21° and 159° with fixedθof 80°, respectively.andare depicted as red and blue arrows inside the hole, respectively. The white arrows represent the direction of the surface current. Figure 1: Calculated field and current distributions around a subwavelength hole. The metal film has been assumed to be a near-perfect electric conductor with a hole diameter of 0.08 λ and a thickness of 0.02 λ . ( a , b ) Normalized electric and magnetic field strength distribution with the normal incidence ( , ), respectively. ( c ) Schematic of setup with an oblique incidence ( θ ≠0°) in the xz plane, with the polarization angle φ . ( d , e ) Surface current distribution on the exit side of the hole for φ =21° and 159° with fixed θ of 80°, respectively. and are depicted as red and blue arrows inside the hole, respectively. The white arrows represent the direction of the surface current. Full size image The best way to separate the effects of electric and magnetic fields on this metallic aperture is to probe the structure with light at oblique incidence angles, having an asymmetric polarization that is neither purely transverse electric (TE, φ =0°) nor transverse magnetic (TM, φ =90°), where φ is the polarization angle ( Fig. 1c ). We consider a detector placed along the z axis and hence insensitive to the normal field components. In this case, the incident electric and magnetic fields projected onto the reflecting plane, and are, in general, not orthogonal, which creates an ideal situation to discriminate the electric and magnetic nature of the scattering. In Figure 1d,e , finite-difference-time-domain (FDTD) calculations of surface currents on the scattering side of the structure, for the case of an oblique incident angle ( θ =80°) with φ =21° and 159°, respectively, are shown, with and depicted by blue and red arrows, respectively. For both the cases, the surface current profile is aligned perpendicular to the tangential magnetic field, with the incident electric field direction seemingly irrelevant. Continuously changing the electric field direction while maintaining a constant magnetic field direction can be achieved by varying the wavevector of the incident light with almost no effect on the surface current distribution. These observations strongly suggest that the surface currents on the scattering side of the structure are of an induced nature, with its symmetric axis determined by the incident magnetic field , where ñ is the unit vector normal to the plane, in our case . With the surface current profile on the scattering side determined primarily by the incident magnetic field, the far-field radiation polarization also reflects the magnetic field direction, at least for the above example of a nearly perfect conductor. As its far-field polarization is invariant with respect to changes in the incident electric field direction because of the negligible tangential electric field on the metal surface, the subwavelength aperture, when combined with far-field polarization analysis, senses the orientation of magnetic vector field. The incident magnetic field direction can be obtained simply by rotating the polarization of the scattered light by 90°. The critical question is whether the surface current profile and radiation polarization of the aperture would still be determined primarily by the incident optical frequency magnetic field in which the metal has less-than-ideal metal conductivities, and when the aperture is larger than the pure quasistatic regime analysed here. Experimental realization of Bethe's magnetic analyser To find out whether a subwavelength hole of these more easily realizable dimensions and materials can still sense the orientation of magnetic vector field, we experimentally investigate the scattering of 780 nm wavelength light by an 80 nm diameter circular aperture in an 80 nm thick gold film deposited on a sapphire substrate. Our strategy to assess the magnetic functionality of the hole relies on identifying the effects of and on the scattering polarization. 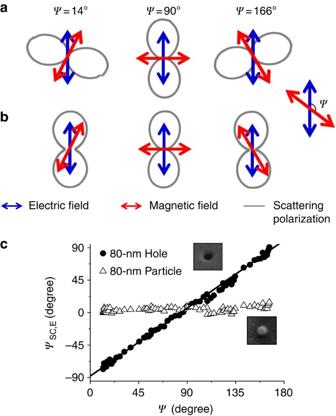Figure 2: Scattering polarization from an aperture and a particle. Measured (λ=780 nm) scattering polarization from an 80-nm aperture and an 80-nm gold nanoparticle. (a) Polar plot (grey) of the scattering polarization for the aperture, and (b) for the nanoparticle with the chosen relative angles (ψ=14°, 90°, 166°) of(red) measured from(blue). (c) The scattering polarization (measured from,ψsc, E) versusψfor the aperture (filled circles) and for the particle (open triangles). Figure 2a shows the polarization analysis of the scattered light on the surface normal direction ( z axis), for three different angles ψ between and . The surface normal scattering angle for the detector is chosen so as to ignore the radiation by z axis dipoles. Strikingly, the scattered polarization is not along , but is perpendicular to , with <5° of deviation. For comparison, we also measure scattering from an 80 nm diameter gold nanoparticle ( Fig. 2b ). For the nanoparticle, a completely opposite behaviour relative to the subwavelength hole is observed with the polarization of scattered light following alone, essentially independent of the optical frequency magnetic field. Figure 2: Scattering polarization from an aperture and a particle. Measured ( λ =780 nm) scattering polarization from an 80-nm aperture and an 80-nm gold nanoparticle. ( a ) Polar plot (grey) of the scattering polarization for the aperture, and ( b ) for the nanoparticle with the chosen relative angles ( ψ =14°, 90°, 166°) of (red) measured from (blue). ( c ) The scattering polarization (measured from , ψ sc, E ) versus ψ for the aperture (filled circles) and for the particle (open triangles). Full size image To confirm that a single hole combined with far-field polarization analysis is indeed a polarization analyser for optical magnetic vector field, we continuously vary ψ , by changing both θ and φ , and analyse the scattered polarization (details provided in the Methods section). Plotted in Figure 2c , in which the direction of is defined as 0°, the measured scattering polarization angle ψ sc, E follows that of , with a slope of 0.997±0.005 (filled circles). Indeed, the polarization of can simply be determined by rotating the measured polarization by 90°, irrespective of . In stark contrast, the nanoparticle (open triangles), showing essentially a zero slope versus magnetic field orientation change, behaves as an electric field analyser [20] , [22] , [32] , [33] , sensitive to only the orientation of electric field. Our results show that from the normal angle scattering off a subwavelength circular aperture, the incident magnetic field can be determined simply by , where is the scattered electric field from the hole. It should be noted that as the size of the hole becomes larger, the scattered polarization begins to align more and more towards , eventually becoming consistent with the prediction of the vector Kirchhoff formalism ( see Supplementary Information ). Flat-bottom NSOM probe for determining magnetic field orientation With a realistic subwavelength aperture on an infinite metal plane behaving as a nanoscale polarization analyser for optical magnetic field, it logically follows to ask whether a circular aperture on a finite-size plane also shows this same behaviour. Recently, it has been shown theoretically that for a certain class of subwavelength optics problems, only a zone of the size ∼ λ /2 (lambda zone) contributes to the scattering, with zones external to this volume contributing negligibly [34] . This raises the intriguing possibility that a flat region of a size ∼ λ /2 surrounding at circular aperture of a metal-coated near-field optical scanning microscopy (NSOM) tip may be sufficient for magnetic functionality, for a straightforward integration of this concept into the existing NSOM technology. 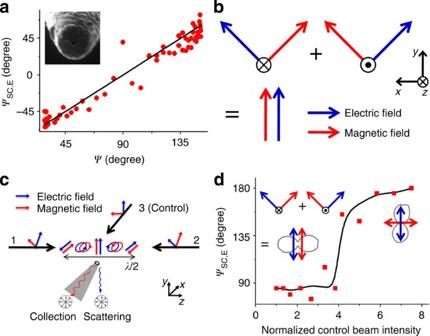Figure 3: Measuring parallel electric and magnetic fields. Measurements (λ=780 nm) of parallel electric and magnetic field polarizations for the demonstration of the magnetic field orientation as an independent entity. (a) The angle of polarizationψsc, Efor the collection signal from a flat-bottomed near-field optical scanning microscopy (NSOM) probe plotted againstψ, showing that this probe is a magnetic field analyser. (b) Schematic for the generation of parallel electromagnetic fields using two counter-propagating, orthogonally polarized light. (c) Experimental schematic for the generation and measurement of parallel electromagnetic fields. Polarization on the probe aperture is controlled by applying an additional phase to beam 1. The collection signal is analysed by a linear polarizer in front of the detector. (d) Experimental control of magnetic field orientation by tuning the intensity of the control beam 3. Polar plots of the representative collection signal (grey) are shown in the inset, showing transition from the parallel electric and magnetic fields case to the normal case of perpendicular electric and magnetic fields. Shown in Figure 3a (inset) is an NSOM probe with a flat apex of about 0.6 λ surrounding a circular aperture of size 0.1 λ ( λ =780 nm), made by focused ion beam milling of an aluminium-coated, etched optical fibre. Figure 3a shows the collection signal polarization ψ sc, E versus ψ , showing a slope of unity, clearly demonstrating that an NSOM probe with a sufficiently large and flat metallic end facet is indeed an analyser for the tangential magnetic field direction. We note that the geometry of the probe apex is crucial in determining which component of light is measured through the probe. Tangential electric or vertical magnetic field [15] , [16] , [17] may be predominantly measured using a metal-coated fibre probe, depending on the shape of the probe apex, such as the precise fraction of flat area on the probe tip; it is noted that an NSOM probe with a circular aperture-sensing vertical magnetic field would produce an unpolarized/circularly polarized light, which is not the case for our tip. Figure 3: Measuring parallel electric and magnetic fields. Measurements ( λ =780 nm) of parallel electric and magnetic field polarizations for the demonstration of the magnetic field orientation as an independent entity. ( a ) The angle of polarization ψ sc, E for the collection signal from a flat-bottomed near-field optical scanning microscopy (NSOM) probe plotted against ψ , showing that this probe is a magnetic field analyser. ( b ) Schematic for the generation of parallel electromagnetic fields using two counter-propagating, orthogonally polarized light. ( c ) Experimental schematic for the generation and measurement of parallel electromagnetic fields. Polarization on the probe aperture is controlled by applying an additional phase to beam 1. The collection signal is analysed by a linear polarizer in front of the detector. ( d ) Experimental control of magnetic field orientation by tuning the intensity of the control beam 3. Polar plots of the representative collection signal (grey) are shown in the inset, showing transition from the parallel electric and magnetic fields case to the normal case of perpendicular electric and magnetic fields. Full size image Measurements of a magnetic field parallel to the electric field A definitive proof of this nanomagnetic field polarization analyser functionality is to test its ability to discern a situation where the electric and magnetic fields of light are aligned in parallel. Another test would be to have a situation with a linear polarized electric field and a circularly polarized magnetic field. These two electromagnetic field configurations can be realized simply by interfering two counter-propagating and two orthogonally propagating beams, respectively. To measure the electric and magnetic field polarizations at a given position on the nanometre scale, two different detection channels of an NSOM probe are used: the orientation of magnetic vector field is determined by the collection signal through an aperture of the probe, whereas the electric polarization is determined by the electric dipole scattering at the apex of the probe [22] , [32] , [33] . Orientations of the electric and the magnetic field are determined by linear polarizers positioned in front of the scattering and collection mode detectors, respectively [32] . We first create mutually parallel local electric and magnetic fields by interfering two counter-propagating beams with orthogonal polarizations (wavelength=780 nm; beams 1 and 2) as shown in Figure 3b . The mathematical expression of the electric and magnetic fields are given by , , respectively. k 0 is defined as the wavevector, and ϕ is defined as the relative phase between beams 1 and 2. By controlling ϕ ( k 0 z + ϕ /2=0 or π), positions at which the electric and magnetic fields are both linearly polarized as well as parallel to each other are created. As shown in Figure 3c , by measuring the polarization resolved collection and scattering signals from an NSOM probe [35] , we identify the position at which the electric field is along the y axis (vertical) where the magnetic field is expected to be parallel to the electric field. Indeed, the magnetic field direction obtained by the collection NSOM is parallel to the electric field ( Fig. 3d , left side inset). Next, we use a control beam (beam 3), gradually increasing its intensity to restore the normal situation where the electric and magnetic fields are perpendicular to each other ( Fig. 3d , right side inset). Our polarization measurements directly show this switching from the unusual situation of parallel electric and magnetic field components to the normal situation of perpendicular field components. Circularly polarized magnetic and linearly polarized electric fields Second, by interfering orthogonally propagating, co-(electrically) polarized beams (beams 1 and 3; wavelength=780 nm), we create a linearly polarized electric field together with a circularly polarized magnetic field ( Fig. 4a ). The mathematical expressions for the electric and magnetic fields along the z axis are given by , , respectively. By varying the relative phase between the two orthogonally propagating beams, the magnetic field is expected to switch between linear ( k 0 z + ϕ ′=0 or π) and circular polarizations ( k 0 z + ϕ ′=π/2 or 3π/2), whereas the electric field polarization is fixed along the y axis ( Fig. 4b ). Indeed, although the scattering signal of the electric field remains essentially linear (blue squares, Fig. 4c right inset), the collection signal of the magnetic field (red squares, Fig. 4c right inset) shows a strong modulation in the polarization linearity, defined as the intensity of the major axis polarization divided by that of the minor axis polarization. Ellipsometric experiments [36] demonstrate that the orientation of magnetic field undergoes a transformation between essentially linear, right-handed and left-handed circularly polarized states with this phase change ( Fig. 4c ). 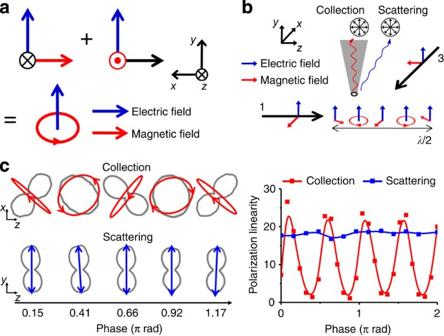Figure 4: Measuring linearly polarized electric and circularly polarized magnetic fields. (a) Schematic for the generation of linearly polarized electric and circularly polarized magnetic fields using two orthogonally propagating light (λ=780 nm). (b) Experimental schematic for the generation and measurement of circularly polarized magnetic field along with linearly polarized electric field. (c) Polar plots for the collection (up) and scattering (down) mode signals. Magnetic field orientation (red) is obtained from the collection near-field optical scanning microscopy (NSOM) signal, via, showing alternation between circularly polarized states and linearly/highly elliptically polarized states. Electric field polarization (blue) remains fixed along theyaxis. Phase-dependent polarization linearity for the scattering and collection signal, in which the polarization linearity is defined as the intensity ratio of major axis polarization and minor axis polarization (right inset). Figure 4: Measuring linearly polarized electric and circularly polarized magnetic fields. ( a ) Schematic for the generation of linearly polarized electric and circularly polarized magnetic fields using two orthogonally propagating light ( λ =780 nm). ( b ) Experimental schematic for the generation and measurement of circularly polarized magnetic field along with linearly polarized electric field. ( c ) Polar plots for the collection (up) and scattering (down) mode signals. Magnetic field orientation (red) is obtained from the collection near-field optical scanning microscopy (NSOM) signal, via , showing alternation between circularly polarized states and linearly/highly elliptically polarized states. Electric field polarization (blue) remains fixed along the y axis. Phase-dependent polarization linearity for the scattering and collection signal, in which the polarization linearity is defined as the intensity ratio of major axis polarization and minor axis polarization (right inset). Full size image To understand why a single subwavelength aperture functions as a Babinet analogue [37] of a nanoparticle, despite the fact that the conductivity at optical frequencies is very low and that the aperture is only partially subwavelength, we invoke the Leontovich boundary condition [38] . Although metals are much poorer conductors in the optical regime than at microwave frequencies, gold and aluminium at near-infrared and visible frequencies still satisfy another condition for a reasonably good metal: δ ; ≪ λ , with the skin depth δ in the order of 10–20 nm. Under this condition, the surface electric field and surface current are primarily determined by the surface magnetic field, and therefore the incident magnetic field: , where ɛ is the dielectric constant of the metal. This is reflected on the scattering side of the subwavelength aperture, enabling it to sense the orientation of magnetic vector field. As the wavelength becomes shorter and | ɛ | gets smaller, the Leontovich boundary condition no longer holds, and the subwavelength aperture would lose its functionality ( Supplementary Methods ); the error would be of the order of 1/| ɛ |. If strong electric dipole sources such as fluorescing quantum dots [39] , [40] or molecules [41] , [42] would exist inside the aperture, the Leontovich boundary condition again would no longer hold and the magnetic functionality would be lost. To conclude, we have shown that normal-angle scattering from a subwavelength aperture in a metal plane is governed by the magnetic field component of light, establishing the aperture as a polarization analyser for magnetic vector field. Magnetic field polarization as an independent physical reality, apart from the electric field polarization, is important when more than one wave vector is present: metamaterials provide specific examples of this, where the magnetic and electric field components are generally neither perpendicular to each other nor equal in strength. This work provides a unique, new optical component for the study of ultrahigh frequency magnetism in metamaterials and other high permittivity materials. Simulation methods Our 3D-FDTD analysis assumed a near perfect electric conductor metal film ( ɛ =−5,000+5,000 i ) with an aperture of 0.08 λ diameter punctured in a metal film thickness of 0.02 λ . A minimum grid size of λ /400 was used after confirming the convergence of the solution as a function of grid resolution. The grid size was gradually increased to λ /20, as the region of interest moved to the far-field region, devoid of any metal structure. For the incident source, a 5 λ ×5 λ -plane wave source was used. Perfectly matched layers of negligible reflectance were also used on the boundary. The surface current density ( K ) distribution on the exit side of the metallic surface was extracted from FDTD-calculated tangential electric field on the metal–surface boundary, following the relation , where σ is conductivity of metal. Experimental data analysis The functionality of the subwavelength aperture as the polarization analyser for optical magnetic field is demonstrated when the effects of electric and magnetic fields on the scattering polarization are identified and compared with a gold nanoparticle. 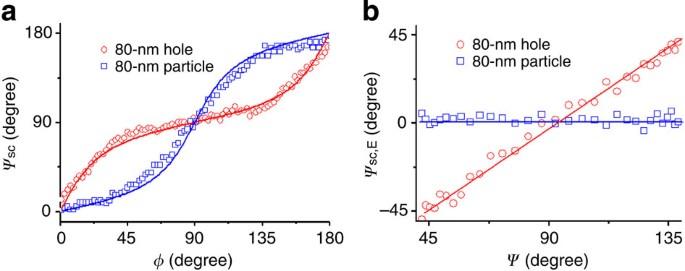Figure 5: Scattering polarizations of a nanohole and a nanoparticle. The scattering polarizations of a nanohole and a nanoparticle are found to follow magnetic field and electric field orientations respectively. (a) Experimentally (λ=780 nm) measured scattering polarization (ψsc) of an 80 nm diameter gold nanoparticle (open blue square) and an 80 nm diameter hole punctured on an 80 nm thick gold film (open red circle). The lines denote fits assuming electric and magnetic dipolar radiations, respectively. (b) Scattering polarization measured from the tangential electric field,ψsc, Eis plotted as a function ofψ. Red and blue lines are linear curves with slope of one and zero, respectively. Following the notations of the experimental schematic depicted in Figure 1c , the scattering polarization ( ψ sc, angle between and x̃ ) for the hole and for the gold nanoparticle as a function of incident polarization ( φ ), are experimentally measured as shown in Figure 5a . The diameters of the hole and particle are both 80 nm, and the incident angle θ is fixed at 70°. Figure 5: Scattering polarizations of a nanohole and a nanoparticle. The scattering polarizations of a nanohole and a nanoparticle are found to follow magnetic field and electric field orientations respectively. ( a ) Experimentally ( λ =780 nm) measured scattering polarization ( ψ sc ) of an 80 nm diameter gold nanoparticle (open blue square) and an 80 nm diameter hole punctured on an 80 nm thick gold film (open red circle). The lines denote fits assuming electric and magnetic dipolar radiations, respectively. ( b ) Scattering polarization measured from the tangential electric field, ψ sc, E is plotted as a function of ψ . Red and blue lines are linear curves with slope of one and zero, respectively. Full size image We first note that the relative angle ψ between and can be expressed as, Then, we obtain the other relative angle ψ sc, E between and from the experimentally measured scattering polarization angle ψ sc . The plot of ψ sc, E versus ψ in Figure 5b shows that the scattering angle follows the orientation of with an offset of ∼ 90° for the hole, whereas the scattering angle by the nanoparticle is fixed along , regardless of the orientation. How to cite this article: Kihm, H. W. et al . Bethe-hole polarization analyser for the magnetic vector of light. Nat. Commun. 2:451 doi: 10.1038/ncomms1430 (2011).